Crystal structure of a common GPCR-binding interface for G protein and arrestin G-protein-coupled receptors (GPCRs) transmit extracellular signals to activate intracellular heterotrimeric G proteins (Gαβγ) and arrestins. For G protein signalling, the Gα C-terminus (GαCT) binds to a cytoplasmic crevice of the receptor that opens upon activation. A consensus motif is shared among GαCT from the G i /G t family and the ‘finger loop’ region (ArrFL1–4) of all four arrestins. Here we present a 2.75 Å crystal structure of ArrFL-1, a peptide analogue of the finger loop of rod photoreceptor arrestin, in complex with the prototypical GPCR rhodopsin. Functional binding of ArrFL to the receptor was confirmed by ultraviolet-visible absorption spectroscopy, competitive binding assays and Fourier transform infrared spectroscopy. For both GαCT and ArrFL, binding to the receptor crevice induces a similar reverse turn structure, although significant structural differences are seen at the rim of the binding crevice. Our results reflect both the common receptor-binding interface and the divergent biological functions of G proteins and arrestins. The G-protein-coupled receptor (GPCR) rhodopsin is composed of a seven transmembrane helix (7-TM) bundle and a covalently attached retinal ligand, which undergoes light-induced isomerization to yield the photoproduct metarhodopsin II and the R* conformation capable of coupling to the G protein transducin (G t ) [1] ( Fig. 1 ). The G t α C-terminus (G t αCT) is disordered in uncomplexed G t but forms an α-helix terminated by a reverse turn (C-cap) upon interaction with the R* cytoplasmic crevice [2] , [3] , [4] , [5] , [6] . Signal transduction is followed by signal shut-off: rhodopsin kinase phosphorylates the R* C-terminus, which recruits rod photoreceptor arrestin for high-affinity interaction with R* (ref. 7 ). Interaction of arrestin with the phosphorylated R* C-terminus displaces the long C-terminal tail (C-tail) of arrestin. As a result, the arrestin basal state, which is structurally similar in all four arrestins [8] , [9] , [10] , [11] , is activated for R* binding ( Fig. 1 ). Insight into the structure of activated arrestin was recently gained by crystal structures of pre-activated C-terminally truncated rod photoreceptor arrestin (p44) [12] or β-arrestin-1 co-crystallized with a synthetic phosphorylated peptide derived from V2 vasopressin receptor C-terminus [13] . In comparison to basal arrestin, pre-activated arrestin shows rearrangements of binding loops in the central crest region, including the so-called finger loop (ArrFL) [14] , [15] , [16] , [17] , [18] , [19] , suggesting that C-tail displacement releases these loops for interaction with R* ( Fig. 1 ). The present work was motivated by the observation of a consensus sequence motif, (E/D)x(I/L)xxxGL, which is conserved in G t αCT and the finger loop of all four arrestins ( Fig. 1 , inset and Supplementary Fig. 1 ). We address the question of how arrestins employ the cytoplasmic crevice within the 7-TM bundle of the active receptor R* for the high-affinity interaction necessary to block G protein binding and/or stimulate arrestin-mediated signalling [13] . Co-crystals of active rhodopsin (R*) with a peptide analogue derived from the finger loop of the rod photoreceptor arrestin (ArrFL-1) were obtained, which diffracted up to 2.75 Å resolution. Similar to G t αCT [3] , ArrFL binds to the cytoplasmic crevice of R* with a C-terminal reverse turn-like structure that involves the conserved E(D)RY motif of R*. Consistently, functional experiments demonstrate similar R*-binding properties of G i /G t and ArrFL peptides. However, in ArrFL-1, the interaction with TM5/6 is partially replaced by interactions with TM7/H8 (specifically the NPxxY(x) 5,6 F motif). We discuss if and how the similarities between GαCT and ArrFL reflect common mechanisms of signal transfer between receptor and interacting proteins. At the same time, the differences between GαCT and ArrFL might indicate the different biological functions of G protein and arrestin. 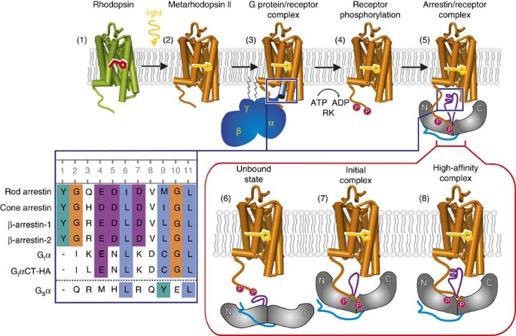Figure 1: Overview of rhodopsin signal transduction and deactivation. (1) Dark-state bovine rhodopsin with inverse agonist 11-cis-retinal. (2) Light-activation and formation of metarhodopsin II (Meta II) with agonist all-trans-retinal. (3) Coupling to the heterotrimeric G protein. (4) Phosphorylation of the activated receptor by its specific kinase. (5) Rod photoreceptor arrestin binding to the phosphorylated receptor. Inset (red box): (6) Basal arrestin approaches phosphorylated Meta II. (7) Interaction with receptor-attached phosphates activates arrestin. (8) Tight binding of the receptor by arrestin (induces further structural changes in arrestin finger loop). Inset (indigo box): Sequence alignment of proposed common sequence motif: rod photoreceptor arrestin (Arr1, residues 68–77), cone photoreceptor arrestin (Arr4, residues 63–72), β-arrestin-1 (Arr2, residues 64–73), β-arrestin-2 (Arr3, residues 65–74), wild-type GtαCT (residues 340–349), high-affinity variant GtαCT-HA (residues 340–349), Gsα (residues 385–394). Figure 1: Overview of rhodopsin signal transduction and deactivation. (1) Dark-state bovine rhodopsin with inverse agonist 11- cis -retinal. (2) Light-activation and formation of metarhodopsin II (Meta II) with agonist all- trans -retinal. (3) Coupling to the heterotrimeric G protein. (4) Phosphorylation of the activated receptor by its specific kinase. (5) Rod photoreceptor arrestin binding to the phosphorylated receptor. Inset (red box): (6) Basal arrestin approaches phosphorylated Meta II. (7) Interaction with receptor-attached phosphates activates arrestin. (8) Tight binding of the receptor by arrestin (induces further structural changes in arrestin finger loop). Inset (indigo box): Sequence alignment of proposed common sequence motif: rod photoreceptor arrestin (Arr1, residues 68–77), cone photoreceptor arrestin (Arr4, residues 63–72), β-arrestin-1 (Arr2, residues 64–73), β-arrestin-2 (Arr3, residues 65–74), wild-type G t αCT (residues 340–349), high-affinity variant G t αCT-HA (residues 340–349), G s α (residues 385–394). Full size image The structure of Ops*–ArrFL-1 We co-crystallized R* (light-activated rhodopsin (Meta II) or the active form of the apoprotein, Ops*) with ArrFL peptides derived from rod photoreceptor arrestin ( 67 YGQEDIDVMGL 77 =ArrFL-1), β-arrestin-1 and β-arrestin-2 ( 63/64 YGREDLDVLGL 73/74 =ArrFL-2/3). Our first strategy was to illuminate a mixture of rhodopsin and ArrFL peptides directly before crystallization ( Supplementary Figs 2 and 3 ). The resulting crystal structures (Meta II–ArrFL) showed weak electron density for both the all- trans -retinal ligand and the peptides (only three residues from the C-terminus were resolved). This problem was most likely due to structural heterogeneity within the crystal, which we overcame by co-crystallizating Ops* and ArrFL peptides. Best results were obtained with ArrFL-1, which diffracted up to 2.75 Å resolution ( Fig. 2 , Table 1 , Supplementary Figs 2–4 ). The Ops*–ArrFL-1 structure contains amino acids 2–326 of opsin, including the 7-TM helices connected by extracellular (EL1–EL3) and cytoplasmic (CL1–CL3) loops, and the cytoplasmic helix 8 (H8), which runs along the membrane surface ( Fig. 2a , Supplementary Fig. 4 ). The last 22 C-terminal amino acids of Ops* were not resolved, presumably due to their high flexibility. The atomic structure of the ArrFL-1 peptide (residues 71–77) was solved from a continuous electron density located within the cytoplasmic crevice of R* ( Supplementary Fig. 4 ), whereas the N-terminal extended part of the peptide (residues 71–73) showed weaker electron density ( Supplementary Table 1 ). Well-defined electron density for a detergent molecule, β- D -octylglucopyranoside, is present within the ligand-binding pocket of R* ( Supplementary Fig. 5 ) [20] . Note that the overall structure of the receptor in all Meta II–ArrFL peptide complexes are essentially the same as the Ops*–ArrFL-1 structure. 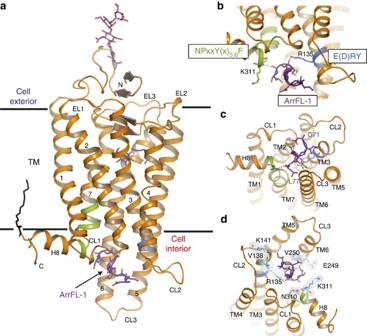Figure 2: Overall structure of the Ops*–ArrFL-1 complex. (a) The active receptor Ops* (orange) and the ArrFL-1 peptide (purple) are shown in ribbon representation, and the ArrFL-1 side chains are shown as sticks. Oligosaccharides at Asn15NT(pink) and a palmitoyl chain at Cys3238.60(black) are presented as sticks. The detergent molecule, β-D-octylglucopyranoside (blue), is shown within the ligand-binding pocket as sticks. (b) Side view and (c) top view of the binding crevice of Ops*. Major hydrogen bonding interactions of Ops* with ArrFL-1 are shown between Leu77 and Lys3118.48from the NPxxY(x)5,6F motif (green), and Met75 and Arg1353.50from the E(D)RY motif (blue). (d) Additional rotated top view of the binding crevice of Ops*. Hydrophobic interactions between ArrFL-1 and residues in the binding interface of Ops* protein moiety are shown as sticks and spheres (light-blue). Arg1353.50of TM3, Val1383.53, Lys141CL2of CL2, Glu2496.32, Val2506.33of TM6 and Asn3108.47, Lys3118.48of TM7/H8 are in van der Waals contact to ArrFL-1 (that is, separated by less than 4 Å). Figure 2: Overall structure of the Ops*–ArrFL-1 complex. ( a ) The active receptor Ops* (orange) and the ArrFL-1 peptide (purple) are shown in ribbon representation, and the ArrFL-1 side chains are shown as sticks. Oligosaccharides at Asn15 NT (pink) and a palmitoyl chain at Cys323 8.60 (black) are presented as sticks. The detergent molecule, β- D -octylglucopyranoside (blue), is shown within the ligand-binding pocket as sticks. ( b ) Side view and ( c ) top view of the binding crevice of Ops*. Major hydrogen bonding interactions of Ops* with ArrFL-1 are shown between Leu77 and Lys311 8.48 from the NPxxY(x) 5,6 F motif (green), and Met75 and Arg135 3.50 from the E(D)RY motif (blue). ( d ) Additional rotated top view of the binding crevice of Ops*. Hydrophobic interactions between ArrFL-1 and residues in the binding interface of Ops* protein moiety are shown as sticks and spheres (light-blue). Arg135 3.50 of TM3, Val138 3.53 , Lys141 CL2 of CL2, Glu249 6.32 , Val250 6.33 of TM6 and Asn310 8.47 , Lys311 8.48 of TM7/H8 are in van der Waals contact to ArrFL-1 (that is, separated by less than 4 Å). Full size image Table 1 Data collection and refinement statistics. Full size table The R* structure presented here is similar to previous structures of active rhodopsin (Ops* or Meta II), alone [4] , [21] or bound to high-affinity variants of the G t αCT peptide [3] , [4] , [22] ( Supplementary Fig. 6 ). The Ops*–ArrFL-1 complex displays the hallmarks of GPCR activation, including the outward tilt of TM6 (>7 Å) and inward motion of TM5, that open the cytoplasmic receptor surface and form a crevice for ArrFL-1 binding. The C-terminal residues 73–77 of ArrFL-1, which were also predicted by mutagenesis as a key binding site with R* (ref. 17 , fold similar to the corresponding section of G t αCT ( Supplementary Fig. 6 ). The conformation of ArrFL-1 is reminiscent of the helical structure predicted by other studies [16] , [23] . The presence of Gly76 facilitates the formation of a reverse turn-like structure, similar to the typical αL-type C-capping motif (C-cap) previously observed for G t αCT [3] ( Supplementary Fig. 6 ). In ArrFL-1, formation of the reverse turn-like structure is made possible by the strong internal hydrogen bonding from Asp73 (main chain carbonyl, MC-O) to Leu77 (main chain amide, MC-N; Fig. 3c ) and the flexibility of Gly76, facilitating a left-handed turn conformation. Despite this similarity, the positioning of ArrFL and G t αCT differ because of the fact that ArrFL is part of a loop connecting two β-strands within arrestin and not the end of a helix like G t αCT. The N-terminal part of ArrFL-1 (residues 71–72) is non-helical and extends in the direction of CL2 of Ops* ( Fig. 2 ). Note that residues 67–70 are not resolved. The structure also indicates that the C-terminal extension of the finger loop would be located between TM6 and TM7/H8. This arrangement would place the cytoplasmic ends of TM1, TM2 and TM7/H8 roughly within the N-domain vestibule of arrestin, whereas the ends of TM3, TM5 and TM6 would be positioned near the central crest of arrestin. 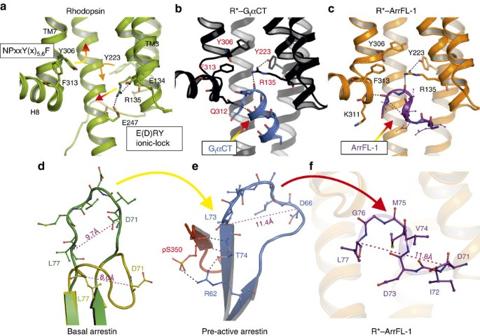Figure 3: The triple role of Arg1353.50and changes in finger loop during arrestin activation and binding. (a) In dark-state rhodopsin (green), the helical bundle is bound together by multiple intra-helical interactions involving the highly conserved E(D)RY and NPxxY(x)5,6F motifs. The arrows indicate side chain motions that occur upon receptor activation. (b) Binding of GtαCT (blue) within the cytoplasmic crevice of R* (black). Main interactions include hydrogen bonding from Arg1353.50to the C-cap, and extensive hydrophobic interactions along the inner face of TM5/TM6. (c) Binding of ArrFL-1 (purple) within the cytoplasmic crevice of R* (orange). Main interactions include hydrogen bonding from Arg1353.50to the reverse turn like structure and Lys3118.48to the GL sequence of ArrFL-1. (d) Finger loop in basal rod photoreceptor arrestin (PDB entry 1CF1) in ‘closed’ (olive) and ‘open’ (dark-green) conformations. (e) Finger loop in β-arrestin-1 (blue) bound to peptide analogue of the phosphorylated receptor C-terminus (red; PDB entry 4JQI). (f) Finger loop peptide ArrFL-1 (purple) bound within the crevice of R*. Ind–f, the backbone Cα-Cα distance between Asp71/67 and Leu77/73 (numbering refers to rod photoreceptor arrestin/β-arrestin-1) is indicated (Å). Figure 3: The triple role of Arg135 3.50 and changes in finger loop during arrestin activation and binding. ( a ) In dark-state rhodopsin (green), the helical bundle is bound together by multiple intra-helical interactions involving the highly conserved E(D)RY and NPxxY(x) 5,6 F motifs. The arrows indicate side chain motions that occur upon receptor activation. ( b ) Binding of G t αCT (blue) within the cytoplasmic crevice of R* (black). Main interactions include hydrogen bonding from Arg135 3.50 to the C-cap, and extensive hydrophobic interactions along the inner face of TM5/TM6. ( c ) Binding of ArrFL-1 (purple) within the cytoplasmic crevice of R* (orange). Main interactions include hydrogen bonding from Arg135 3.50 to the reverse turn like structure and Lys311 8.48 to the GL sequence of ArrFL-1. ( d ) Finger loop in basal rod photoreceptor arrestin (PDB entry 1CF1) in ‘closed’ (olive) and ‘open’ (dark-green) conformations. ( e ) Finger loop in β-arrestin-1 (blue) bound to peptide analogue of the phosphorylated receptor C-terminus (red; PDB entry 4JQI). ( f ) Finger loop peptide ArrFL-1 (purple) bound within the crevice of R*. In d – f , the backbone Cα-Cα distance between Asp71/67 and Leu77/73 (numbering refers to rod photoreceptor arrestin/β-arrestin-1) is indicated (Å). Full size image ArrFL-1 forms specific contacts with two highly conserved motifs in the receptor: Arg135 3.50 within E(D)RY and Lys311 8.48 within NPxxY(x) 5,6 F ( Fig. 2; note: superscript following residue number refers to Ballesteros–Weinstein numbering, see Full Methods). A hydrogen bond (distance 2.85 Å) is formed between Met75 (MC-O) of ArrFL-1 and the guanidine group of Arg135 3.50 in R* ( Figs 2b and 3c , Supplementary Figs 7, 8 and 11 ). This bond is similar to that observed for Cys347 in G t αCT and Arg135 3.50 ( Fig. 3b ). Lys311 8.48 within the NPxxY(x) 5,6 F motif forms a distinct hydrogen bond with ArrFL-1: Lys311 8.48 (MC-N) to Gly76 (MC-O) (distance 2.97 Å; Figs 2b and 3c , Supplementary Figs 7, 8 and 11 ). In contrast, Gln312 8.49 (side chain) makes a hydrogen bond with Lys345 (MC-O) of G t αCT ( Fig. 3b , Supplementary Figs. 7 and 8 ). Both ArrFL-1 and G t αCT are in van der Waals contact with Asn310 8.47 ( Fig. 2d , Supplementary Figs 7 and 8 ). Note that no strong interactions of polar side chains of ArrFL-1 with the receptor are visible. Furthermore, additional van der Waals contacts are formed between Ile72 on ArrFL-1 and Val138 3.53 and Lys141 CL2 . In comparison, G t αCT makes contacts with Val138 3.53 , Val139 3.54 and Lys141 CL2 . Overall, the contacts observed between ArrFL-1 and the receptor loops are consistent with previous studies implicating receptor loops CL1 and CL2 in arrestin binding [19] , [24] , [25] , [26] . With respect to receptor binding, the main difference between ArrFL-1 and G t αCT is the contribution of TM5/6. ArrFL-1 makes only minor contacts to TM6 (Leu77 to Glu249 6.32 , Val250 6.33 ) and no contacts to TM5. In contrast, extensive hydrophobic interactions exist between several amino acid side chains of G t αCT (Ile340, Leu341, Phe350) and the ‘hydrophobic wall’ formed by TM5 (Leu226 5.61 , Val230 CL3 , Ala233 CL3 ) and TM6 (Thr242 CL3 , Thr243 CL3 , Ala246 6.29 , Val250 6.33 ; Supplementary Fig. 7 ). In essence, the interactions of ArrFL-1 with TM5/6 are reduced as compared with G t αCT, but those with TM7/H8 (NPxxY(x) 5,6 F motif) and TM3 (E(D)RY motif) are preserved ( Fig. 3c and Supplementary Fig. 8 ). This finding is consistent with recent studies localizing G-protein- and arrestin-specific binding determinants to TM6 and TM7/H8, respectively [27] , [28] , [29] . Functional characterization of peptides To verify the functional relevance of the observed peptide binding to the receptor crevice ( Fig. 4a, b ), we applied three different well-established functional assays. These assays were performed in native disc membranes and not the detergent system used for crystallization, as the native membrane offers many advantages to observe the interactions of peptides with the different functional forms of rhodopsin. In the first assay, we light-activated rhodopsin under conditions favouring Meta I, the inactive precursor of the active species Meta II. Meta I and Meta II can be differentiated by ultraviolet-visible absorption spectroscopy due to their different absorbance maxima. Like both full-length rod photoreceptor arrestin (ref. 30 ) and G t αCT [31] , ArrFL-1 stabilized the 380-nm-absorbing Meta II species over Meta I, showing that ArrFL-1 functionally binds the active state of the receptor. Titration analysis indicated K D values of 2.4 μM and 0.8 mM for G t αCT-HA (high-affinity version) and ArrFL-1, respectively ( Fig. 4c, d ). For comparison, the K D values of the wild-type G t αCT and ArrFL-2/3 are 0.18 and 1.3 mM, respectively ( Supplementary Fig. 9 ). In the second assay, we measured the ability of G t αCT and ArrFL peptides to compete against full-length rod photoreceptor arrestin for binding to phosphorylated opsin (OpsP) in membranes ( Fig. 4e,f , Supplementary Fig. 9 ). The competition data yield K D values of 320 μM, 880 μM, 1.7 mM and 2.4 mM for peptides G t αCT-HA, wild-type G t αCT, ArrFL-1 and ArrFL-2/3, respectively. Importantly, these data indicate that full-length rod photoreceptor arrestin and ArrFL have a common receptor-binding site. The peptide derived from G s αCT from the G s family, which does not share the common sequence motif with ArrFL and G t αCT, did not stabilize Meta II and showed no competition for arrestin binding to phosphorylated opsin ( Supplementary Fig. 9 ). In the third assay, Fourier transform infrared (FTIR) spectroscopy was used to monitor the effects of Meta II–ArrFL-1 complex formation in native membranes resulting in characteristic bands, which mostly appear in the structurally sensitive amide I and amide II regions of the FTIR spectrum [32] , [33] ( Supplementary Fig. 10 ). The effect of ArrFL-1 and ArrFL-2/3 on the R* characteristic difference spectrum is similar to G t αCT, although the data suggest a somewhat smaller influence on the peptide structure due to binding [32] . The G s αCT shows essentially no effect on the difference spectrum, in accordance with its lack of binding in the other assays. In further FTIR experiments, we investigated the R135L mutant and its capability of binding ArrFL-1 peptide ( Supplementary Fig. 10 ). We observed that the characteristic arginine bands are missing upon binding, which suggest an involvement of Arg135 in ArrFL-1 binding under these conditions. Altogether, FTIR data confirm that peptides with the consensus sequence (E/D)x(I/L)xxxGL specifically bind and stabilize the active conformation of the receptor in a very similar manner as G t αCT. It remains to be determined whether, like G t αCT, ArrFL-1 discriminates between different conformational substates of Meta II (ref. 33 ). 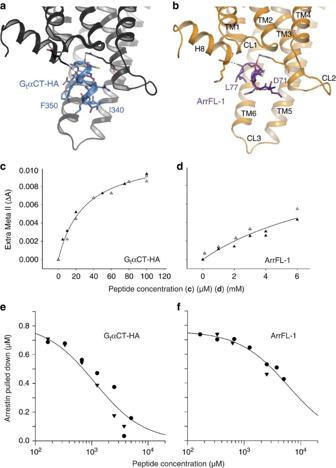Figure 4: Structural and functional comparison of GtαCT and ArrFL-1. (a) Side view of the active receptor Ops* crevice (black ribbons and sticks) with bound GtαCT-HA peptide (blue ribbon and sticks; PDB entry 3DQB). (b) Side view of the active receptor Ops* crevice (orange ribbons and sticks) with bound ArrFL-1 peptide (purple ribbon and sticks). (c) Stabilization of Meta II by the high-affinity peptide GtαCT-HA and (d) ArrFL-1 peptide. (e) Competition against rod photoreceptor arrestin for binding to phosphorylated opsin by GtαCT-HA and (f) ArrFL-1 peptide. In panelsc–f, data points from independent experiments are represented as differently shaped symbols. The peptide titration experiments which measure Meta II-stabilization (c,dandSupplementary Fig. 9a,b,c) yield an apparentKD, from which the trueKDvalue of peptide binding to Meta II can be derived. Further experimental details are given in the Methods. Figure 4: Structural and functional comparison of G t αCT and ArrFL-1. ( a ) Side view of the active receptor Ops* crevice (black ribbons and sticks) with bound G t αCT-HA peptide (blue ribbon and sticks; PDB entry 3DQB). ( b ) Side view of the active receptor Ops* crevice (orange ribbons and sticks) with bound ArrFL-1 peptide (purple ribbon and sticks). ( c ) Stabilization of Meta II by the high-affinity peptide G t αCT-HA and ( d ) ArrFL-1 peptide. ( e ) Competition against rod photoreceptor arrestin for binding to phosphorylated opsin by G t αCT-HA and ( f ) ArrFL-1 peptide. In panels c – f , data points from independent experiments are represented as differently shaped symbols. The peptide titration experiments which measure Meta II-stabilization ( c , d and Supplementary Fig. 9a,b,c ) yield an apparent K D , from which the true K D value of peptide binding to Meta II can be derived. Further experimental details are given in the Methods. Full size image By the common (E/D)x(I/L)xxxGL motif, two structurally and functionally distinct proteins, G protein and arrestin, can recognize similar activation signatures of R* within the E(D)RY and NPxxY(x) 5,6 F motifs. In the case of G protein, GαCT binds within the cytoplasmic crevice of R*, and this information is communicated down the long α5 helix of Gα to the nucleotide-binding site, where GDP/GTP exchange occurs [1] . Recent work has suggested that the flexibility of G t αCT allows it to rapidly enter the binding crevice, and after a process of mutual conformational adaptation, both G t αCT and the cytoplasmic crevice of the receptor gain a well-defined structure [33] . Our data indicate that arrestin partially mimics this process. The finger loop is highly flexible in basal arrestin [8] , [15] , [16] , [18] , [23] , and interaction with the binding crevice of R* induces structuring in the form of a reverse turn. Comparison of crystal structures shows how the finger loop elongates in the progression of arrestin activation from basal to pre-activated to R*-bound ( Fig. 3d–f ). During arrestin activation, the phosphorylated receptor C-terminus forms an extended β-sheet with strand VI near the finger loop, which is held in place by hydrogen bonding to two phosphate moieties ( Fig. 3e ) [13] . This initial interaction of arrestin with the phosphorylated receptor could stabilize and orient the flexible finger loop for tight binding to the crevice of R*. Formation of the high-affinity complex pulls the finger loop further apart and may partially melt the β-sheet composed of strands V and VI. This transformation allows arrestin to block access of G protein to the receptor (signal shut-off) and may also induce other changes in the arrestin protein that promote scaffolding of signalling proteins (arrestin-mediated signalling). In summary, the remarkable homology seen between GαCT and ArrFL suggests that the (E/D)x(I/L)xxxGL motif evolved in both G protein and arrestin to allow recognition and interaction with the same binding crevice presented by the active GPCR. In spite of these similarities, we also identify pronounced differences, namely a larger hydrophobic interaction surface in the case of G t αCT, which may contribute to the distinct biological functions of G proteins and arrestins. Peptide synthesis All peptide experiments in this study were verified at least twice with peptide lots from two different manufacturers (Selleckchem and GenScript). Peptides from Selleckchem and GenScript were purchased with 95% purity as verified by analytical high-performance liquid chromatography and Tandem Mass Spectrometry. Peptides of rod photoreceptor arrestin ( 67 YGQEDIDVMGL 77 , ArrFL-1), β-arrestin-1/2 ( 63/64 YGREDLDVLGL 73/74 , ArrFL-2/3), wild-type G t α ( 340 IKENLKDCGLF 350 , G t αCT) and the high-affinity version of G t α ( 340 ILENLKDCGLF 350 , G t αCT-HA) were synthesized without any modifications. The G s α peptide ( 384 QRMHLRQYELL 394 , G s αCT) was synthesized with or without N-terminal acetylation, which showed no difference in experiments. Purification and crystallization of complexes Rod outer segment (ROS) disc membranes containing rhodopsin were isolated from frozen bovine retina by a multi-step sucrose density gradient centrifugation procedure [34] . All procedures were carried out under dim red light, and retinas were sourced from a local slaughterhouse. Opsin was generated by exposing the isolated ROS membranes to a bright orange light in the presence of hydroxylamine. Membranes containing rhodopsin or opsin were stripped of peripheral proteins by washing three times with 4 M urea [21] , [35] . Stripped membranes were subsequently solubilized in buffer A (20mM 1,3-Bis[tris(hydroxymethyl) methylamino]propane, pH 7.5, 1.25% n-octyl-b- D -glucoside) at a concentration of about 200 μM receptor. All peptides were solubilized in buffer A and the final pH was readjusted to 7.5. Synthetic peptides were added at a 12:1 molar ratio of peptide to protein (final receptor concentration ~150 μM). Rhodopsin/peptide mixtures were kept on ice for 5 min and illuminated (530 nm) for 60 s. The protein/peptide mixtures were crystallized in sitting drops by vapour diffusion at 277 K using 24-well Limbro and 96-well MRC plates. The protein-to-reservoir-solution-ratio was optimized from 1:0.1 to 1:2 using a Mosquito crystallization robot (TTP Labtech). The reservoir solution contained 3.2–3.5 M (NH 4 ) 2 SO 4 in 0.1 M 2-( N -morpholino)ethanesulfonic acid or sodium acetate at pH 6.0. Crystals appeared within 7 days and grew for a further 5 days to reach dimensions 0.3 × 0.3 × 0.4 mm 3 . Crystals were then transferred under red light to cryoprotectant consisting of 10–15% trehalose in crystallization buffer and immediately frozen in liquid nitrogen. Ultraviolet-visible absorption spectra of the crystals were measured offline before X-ray irradiation at 100 K using a HR2000 (OceanOptics) on a microspectrophotometer setup at beamline ID29S (ESRF) [36] ( Supplementary Fig. 2 ). Data collection and structure analysis Diffraction data collections of more than 500 crystals were performed at 100 K using synchrotron X-ray sources from ESRF and BESSY II. The best diffraction data for the highest resolution of Ops*–ArrFL-1 was collected at synchrotron beamline ID29 (ref. 37 ) at ESRF with a Pilatus 6 M detector at 0.9791, nm wavelength. The crystal-to-detector distance was fixed at 521 mm for Ops*–ArrFL-1. All images were indexed, integrated and scaled using the XDS programme package [38] and the CCP4 programme SCALA [39] , [40] . Ops*–ArrFL-1 crystals belonged to the rhombohedral space group H32 (for Ops*–ArrFL-1: a =242.62 Å, b =242.62 Å, c =110.22 Å, α =90°, β=90°, γ =120°). Table 1 summarizes the statistics for crystallographic data collection and structural refinement. Initial phases for Ops*–ArrFL-1 were obtained by the conventional molecular replacement protocol (rotation, translation, rigid-body fitting) using the Ops*–G t αCT structure (PDB accession 3DQB [3] ) without G t αCT peptide as the initial search model, which was used in the programme Phaser [41] . A simulated annealing procedure with the resulting model was performed using a slow-cooling protocol and a maximum likelihood target function, energy minimization and B-factor refinement by the programme PHENIX [42] , which was carried out in the resolution range of 40.04–2.75 Å for the Ops*–ArrFL-1 structure. After the first round of refinements, the ArrFL-1 peptide and β- D -octylglucopyranoside in the ligand-binding pocket were clearly visible in the electron density of both σ A -weighted 2 F o − F c maps, as well as in the σ A -weighted simulated annealing omitted density maps for Ops*–ArrFL-1. Ops*–ArrFL-1 was modelled with TLS refinement [43] (TLS - for Translation, Libration (small movements) and Screw-rotation of a group of atoms) using anisotropic temperature factors for all atoms. Restrained, individual B-factors were refined, and the crystal structure was finalized by the CCP4 programme REFMAC5 (ref. 44 ) and other programmes of the CCP4 suite [39] . The final model has agreement factors R free and R cryst of 25.1 and 21.7%, for Ops*–ArrFL-1. Manual rebuilding of the Ops*–ArrFL-1 model and electron density interpretation were performed after each refinement cycle using the programme COOT [45] . Structure validation was performed with the programmes PHENIX [42] , SFCHECK [46] , PROCHECK [47] , WHAT_CHECK [48] and RAMPAGE [49] . Potential hydrogen bonds and van der Waals contacts were analysed using the programmes HBPLUS [50] and LigPlot+ (ref. 51 ). All crystal structure superpositions of backbone α-carbon traces were performed using the CCP4 programme LSQKAB [39] . All molecular graphics representations in this work were created using PyMol [52] . Superscripts following receptor residue numbers denote N -terminus (NT), Helix 8 (H8), cytoplasmic loop and GPCR numbering according to Ballesteros and Weinstein [53] . The most conserved residue in a helix among rhodopsin-like GPCRs is designated x .50, where x is the helix number. All other residues on the same helix are numbered relative to this reference residue. Spectroscopic analysis of peptide binding ROS membranes containing phosphorylated rhodopsin were prepared from frozen bovine retina (W.L. Lawson Company). Briefly, ROS membranes were isolated using a multi-step sucrose density centrifugation procedure. Phosphorylation of the rhodopsin by the associated native rhodopsin kinase was achieved by exposing the ROS to white light in the presence of adenosine triphosphate (8 mM) and MgCl 2 (2 mM). After 2 h, hydroxylamine (20 mM) was added to convert all rhodopsin photoproducts to opsin. The membranes containing phosphorylated opsin (OpsP) were then washed several times to remove the hydroxylamine and peripheral proteins and finally regenerated with 11- cis -retinal. These procedures have been recently described in detail [54] . Peptides were solubilized in 100 mM HEPES buffer, and the final pH was adjusted to 8.0. ‘Extra Meta II’ analysis was performed at 0 °C using a Shimadzu UV3000 instrument [30] . Note that all peptides used for crystallization were first functionally verified by the absorbance ‘Extra Meta II’ assay. Samples consisted of 10 μM ROS-P in 100 mM HEPES buffer pH 8.0 and increasing concentrations of peptide. The photo-flash activated ~20% of the rhodopsin. The titration data were fit to the expression ( B max * x / K D + x ), where the final amplitude of the plots was fixed to the theoretical maximum absorbance change (that is, 100% Meta II stabilization). The resulting apparent K D value was corrected for Meta I/Meta II equilibrium at pH 8.0 (refs 30 , 55 ). The true K D value of peptide binding to Meta II was derived from the apparent K D value, as described by Schleicher et al. [30] , [55] , using a Meta II/Meta I ratio of ~0.1 (refs 30 , 55 ). Centrifugal pull-down binding assay The preparation of phosphorylated opsin from ROS membranes is described in the method section ‘Spectroscopic analysis of peptide binding’. The bovine rod photoreceptor arrestin mutant C63A/C128S/C143A/W194F/A366C was expressed in E. coli and purified using two-step ion exchange chromatography (heparin and Q sepharose, GE Helathcare Life Sciences) [56] , [57] . This single-cysteine mutant (50 μM) was labelled with a tenfold molar excess of N , N ′-dimethyl- N -(Iodoacetyl)- N ′-(7-Nitrobenz-2-Oxa-1,3-Diazol-4-yl)Ethylenediamine (NBD, Life Technologies) for 3 h at room temperature. Free label was removed by buffer exchange using centrifugal concentrators followed by size exclusion chromatography (Sephadex G-15, 500 μl void volume). NBD-labelled arrestin A366C (A366NBD) is functionally equivalent to wild type [58] . Peptides were solubilized in 50 mM HEPES buffer, and the pH was adjusted to 7.0. Peptide competition against arrestin A366NBD (1 μM) for binding to OpsP (2 μM) was measured by a centrifugal pull-down assay (50 mM HEPES, pH 7.0, 22 °C) [54] , [58] . Briefly, arrestin and OpsP were mixed with increasing concentrations of peptide (120 μl sample volume). Following an equilibration period of ~30 min, samples were centrifuged at 16,000 g for 10 min (room temperature). The absorbance spectrum of each supernatant was then measured. Given the red-shifted absorbance of the NBD label ( λ max =500 nm) and its defined extinction coefficient (0.025 μM −1 cm −1 ), the concentration of arrestin remaining in the supernatant could be accurately determined. The K D of peptide binding to OpsP was determined by fitting the peptide titration data to the expression: y = s *(1–( P /( P + K Dp *(1+ A / K Da ))), where P is the peptide concentration, K Dp is the K D of the peptide, A is the arrestin concentration (1 μM), K Da is the K D of arrestin binding to OpsP (400 nM) [54] . The scaling factor s was necessary as y axis values were not normalized. FTIR spectroscopy FTIR difference spectroscopy is a sensitive monitor of the structural influence of peptide binding on the active receptor [32] , [33] . Briefly, FTIR difference spectra of rhodopsin (~1 mM) were recorded at room temperature and pH 5.8 to ensure exclusive formation of the active receptor conformation upon illumination ( λ max =532 nm). A separate measurement was performed under identical conditions but in the presence of an excess of peptide (5 mM for G t αCT, 14 mM for all other peptides). The peptide binding spectra (difference of the difference spectra recorded in the presence and absence of peptide) were calculated after normalization of all spectra to the difference bands between 1,500 and 1,300 cm −1 . Similar FTIR measurements were carried out for the R135L receptor mutant and the ArrFL-1 peptide. Mutant rhodopsin was expressed in COS-1 cells using the eukariotic expression vector pMT4 (refs 59 , 60 ). After regeneration with 30 μM 11- cis -retinal the protein was purified in 1% n - D -octyl-b- D -glucopyranoside using the 1D4 antibody bound to sepharose resin. Rhodopsin was eluted from the resin with rhodopsin-derived C-terminal peptide 340–348. The protein was thereafter incorporated into egg-PC lipid vesicles at a ratio of 1:100 (rhodopsin/lipid) by dialysis against 20 mM bis-tris propane, 130 mM NaCl, 1 mM MgCl 2 , pH 7.0 (ref. 61 ). Accession codes: The atomic coordinates and structure factors have been deposited in the Protein Data Bank under accession code 4PXF . How to cite this article : Szczepek, M. et al. Crystal structure of a common GPCR-binding interface for G protein and arrestin. Nat. Commun. 5:4801 doi: 10.1038/ncomms5801 (2014).